Threat of invasive pests from within national borders Predicting and ranking potential invasive species present significant challenges to researchers and biosecurity agencies. Here we analyse a worldwide database of pest species assemblages to generate lists of the top 100 insect pests most likely to establish in the United States and each of its 48 contiguous states. For the United States as a whole, all of the top 100 pest species have already established. Individual states however tend to have many more 'gaps' with most states having at least 20 species absent from their top 100 list. For all but one state, every exotic pest species currently absent from a state's top 100 can be found elsewhere in the contiguous United States. We conclude that the immediate threat from known invasive insect pests is greater from within the United States than without. Our findings have potentially significant implications for biosecurity policy, emphasizing the need to consider biosecurity measures beyond established national border interventions. Invasive species cause immense environmental and economic damage worldwide [1] , [2] , [3] , [4] , [5] . In the United States, introduced species are estimated to cost the economy approximately US$120 billion per year [6] , whereas in Europe costs have been estimated at US$13 billion per year [3] . Accordingly, predicting the identity and entry pathway of alien invasive species is of considerable importance for researchers and policy-makers and many countries maintain active biosecurity infrastructures, backed up by national and international regulatory institutions and agreements [7] aimed at preventing introductions of alien invasive pests, weeds and diseases (for example, for the United States, see http://www.csrees.usda.gov/nea/ag_biosecurity/ag_biosecurity.cfm ). Given the increasingly global nature of transport and trade, together with the fact that there are hundreds or even thousands of potential invasive species in the global species pool, a major challenge for national biosecurity is predicting which invasive species are of greatest threat [3] , [8] , [9] and from where those species are likely to come [3] , [10] . In addition, for large countries with multiple potential entry points, there is a need to consider not only pre-border incursions, but also post-border spread of exotic species that have already arrived [3] , [11] , [12] . The current approach of biosecurity agencies to these issues often relies heavily on a consultative process in which scientific experts, policy officers and industry stakeholders are consulted for their opinion on which of the potential invasive species have the highest likelihood of invading. [3] , [13] . However, it is well known that such opinions are susceptible to context dependence and motivational bias, potentially resulting in misleading prioritization [14] and making it difficult to rank and prioritize potentially hundreds of species for different biosecurity contexts (for example, pre- versus post-border, state or regional versus national, agricultural versus environmental). Alternately, there are numerous quantitative approaches to estimating a species likely exotic range, [15] , [16] , [17] , [18] but these require extensive and detailed data regarding a species and/or the environmental characteristics of its range, and are generally completed on a species by species basis (though there are some notable exceptions, which have assessed multiple species [19] , [20] ). To rank and prioritize hundreds of species using any of these approaches would require significant time and cost. Here we apply a type of artificial neural network (a self organizing map or SOM), analysing presence/absence data to rank simultaneously, based on establishment likelihood, the threat of a globally distributed set of >800 known invasive insect pest species to the United States [21] , [22] (data extracted from the CABI Crop Protection Compendium [23] ). The SOM identifies similarities in species assemblages in different regions and then ranks species according to their 'likelihood' of establishing in a particular region based on these species associations. By considering that species groupings are non-random, any species commonly found with a particular set of other species is more likely to establish in a region where elements of that species assemblage are found. This SOM approach therefore captures, phenomenologically, the anthropogenic, biotic and abiotic factors that determine the make up and distribution of species assemblages [21] , [22] , [24] , [25] and presents an alternative to all other current species prioritization processes. We used the SOM approach to analyse the CABI pest data set and generate top 100 'likelihood of establishment' lists for the contiguous USA and for the 48 contiguous states (that is, not including geographically separated Hawaii or Alaska). For each state we then determined whether species absent in their top 100 potential invaders were absent from the United States overall, or could be found already in another US state. The aim was to determine where the greatest current threat from known invasive insect pests lies—within the United States or without? We found that for all but one US state, all absent species in a state's top 100 can be found somewhere else in the contiguous USA, and often in a neighbouring state that shares a border. We conclude that for the United States, the greatest threat from known invasive species comes from within the United States itself rather than from outside. Top 100 lists Our initial analysis revealed a key finding: of the top 100 insect species predicted to have the highest chance of establishment in the United States as a whole ( Supplementary Data 1 ), all are currently present somewhere within the contiguous United States (and 178 of the top 200 are present). Using the top 100 likelihood lists for all 48 states ( Supplementary Data 1 ), we determined how many of the top 100 are still absent from a particular state ( Fig. 1a ). In contrast to the national likelihood list, we found that all states had species absent in their top 100 list, with most states having at least 20 absent species in their top 100 and one state (Vermont) having almost half of the 100 absent (48). 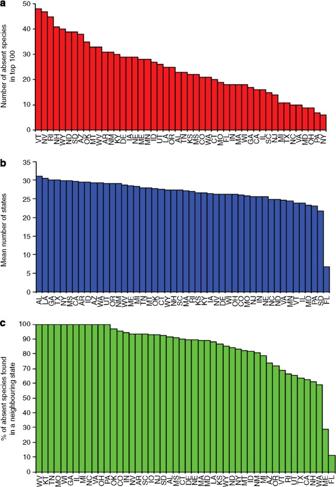Figure 1: Characteristics of each US state's top 100 list. (a) Number of absent species in the top 100 likelihood list for each state of the contiguous USA.(b)Mean number of other states in the contiguous USA an absent species in the top 100 likelihood list is found (e.g. for Alabama, the 23 absent species in its top 100 likelihood list are found, on average, in 31 other states).(c)Percentage of absent species in a state's top 100 likelihood list found in at least one neighbouring state. Figure 1: Characteristics of each US state's top 100 list. ( a ) Number of absent species in the top 100 likelihood list for each state of the contiguous USA. (b) Mean number of other states in the contiguous USA an absent species in the top 100 likelihood list is found (e.g. for Alabama, the 23 absent species in its top 100 likelihood list are found, on average, in 31 other states). (c) Percentage of absent species in a state's top 100 likelihood list found in at least one neighbouring state. Full size image We then asked, of those absent species in a state's top 100 list, how many are present in another state in the United States? In all but one of the 48 contiguous states of the United States, every absent species in the top 100 for a state could be found in at least one other state and on average will be found in 27 other states ( Fig. 1b ). Moreover, we found the majority of absent species in any state's top 100 can be found in a neighbouring state that shares a border ( Fig. 1c ). On average, 84.3% of the absent species could be found in at least one neighbouring state, with 12 states having all absent species in their top 100 present in a neighbouring state ( Fig. 1c ). The only exception to this was Florida, for which 9 out of the 18 species absent in its top 100 are not found anywhere else in the contiguous USA, and a further three species are only found in one other state. Factors related to top 100 lists In determining what factors could predict whether a state has a large number of absent species in the top 100, it might be expected that larger states would accumulate more species than smaller states and therefore have fewer absent species. However, we found no relationship between the number of absent species in a state and state size (linear regression, F 1,46 =0.06, P =0.800; asymptotic regression, F 1,45 =0.76, P =0.476; data presented in Supplementary Fig. S1 ). Similarly, species diversity tends to decrease with latitude [26] so it might be expected that southern states would have fewer absent species than northern states, but again there was no significant relationship between the number of absent species in a state's top 100 and the state latitudinal midpoint (linear regression, F 1,46 =2.50, P =0.121; asymptotic regression, F 1,45 =1.42, P =0.253; data presented in Supplementary Fig. S2 ). In contrast, there was a significant negative relationship with the number of inbound domestic air passengers (asymptotic regression–exponential curve, F 2,45 =12.46, P <0.001, R 2 =0.328; Fig. 2a ), and also gross state product (GSP) (asymptotic regression–exponential curve, F 2,45 =43.45, P <0.001, R 2 =0.644; Fig. 2b ). 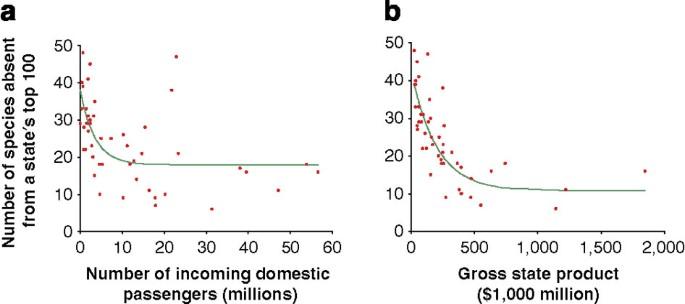Figure 2: Factors related to a US state's top 100 list. (a) Relationship between the number of incoming domestic flight passengers to a state and the number of absent species in that state's top 100 list (fitted curve: 17.96 + 20.04 × 0.749X).(b)Relationship between the gross state product and the number of absent species in that state's top 100 list (fitted curve: 10.81 + 31.96 × 0.995X). Figure 2: Factors related to a US state's top 100 list. ( a ) Relationship between the number of incoming domestic flight passengers to a state and the number of absent species in that state's top 100 list (fitted curve: 17.96 + 20.04 × 0.749 X ). (b) Relationship between the gross state product and the number of absent species in that state's top 100 list (fitted curve: 10.81 + 31.96 × 0.995 X ). Full size image The combined evidence that the United States as a whole has no species absent in its top 100 list and that most absent species in a state's top 100 can be found in a neighbouring state leads to the conclusion that the immediate present-day threat from known invasive insect pests is greater from within the United States than without. Although the SOM analysis does not indicate the likelihood of a pest species actually arriving from a particular state, the fact that species absent from one state were frequently found in a neighbouring state implies the ease at which that pest could arrive. Interestingly, Florida was the only state with absent species in its top 100 that were not found in any other state. The immediate threat from outside the United States may be proportionately greater for Florida than any other contiguous US state. Of all inspection stations at US ports of entry (airports, maritime ports and land border sites), Miami had the greatest percentage (21.8%) of insect interceptions [27] indicating that it receives a significant number of insect pests and may be a 'doorway' to insect pests entering the United States. Inbound domestic passengers and GSP can be considered surrogates for propagule pressure and ecological disturbance respectively [28] , both of which have been identified as determinants of species invasion in other contexts [28] , [29] , [30] , [31] . In line with this, transport ('propagule pressure') and economic activity ('disturbance') appear to be factors in determining the likelihood of establishment of known invasive crop pests in the US states. That is, those states that have a small number of absent species in their top 100 (as determined by the SOM analysis) tend to have higher levels of incoming air passengers (propagule pressure) and higher GSP (ecological disturbance). Another factor that could also determine likelihood of a species being present or absent in a given state is time since arrival and establishment in the United States. However, the reliability of these type of data is notoriously poor (invaders can remain undetected for many years and reporting varies with commodity, surveillance systems, economic significance, feeding ecology, taxonomy and so on) [32] , making systematic analysis difficult. Beyond enabling us to generate likelihood lists for each of the US states, as mentioned in the methods, those regions that are closest together in a SOM, and in particular that share the same neuron, are most similar to one another [21] , [22] , [24] , [33] . Examining which states have been assigned to the same neuron in the current analysis, therefore, reveals which states have the most similar insect pest assemblages ( Fig. 3 ). The insect pest assemblage of a state captures a significant proportion of biological, ecological and abiotic factors that cannot be measured, and states with similar assemblages therefore share these characteristics. Species that are subsequently found in one state would have a high likelihood of establishing in a SOM identified closely clustered state [21] , [22] . The analysis identifies several clusters of states that do show some similarities with regional ecosystem divisions ( http://www.fs.fed.us/land/ecosysmgmt/colorimagemap/ecoreg1_divisions.html ). However, the clusters do not simply follow regional groupings of contiguous states, with some states clustering across very broad regions and others clustering with just one, or even no other states. In terms of invasive species risk and possible biosecurity responses, states within the same cluster are the most likely potential sources of high-establishment pests for one another (a conclusion that should apply to plant pest species in general, not only those species contained within the current pest database) [21] , [22] . This does not mean that states outside an immediate cluster cannot act as sources for insect pest species, but does provide some insights for informing potential biosecurity/phytosanitary measures between states. Whether addition of further invasive species would help provide greater resolution within and between clusters is unclear. However, adding other plant 'pests', such as fungal pathogens, would integrate the influence of other taxa and could be valuable to biosecurity agencies that need to consider all potential threats to crops. However, the addition of non-plant pests that occupy fundamentally different niches (for example, pests of native systems) could weaken the inferences with respect to agriculture (although it would be interesting to conduct separate SOM analyses to explore emergent patterns and resultant biosecurity implications for different classes of invasive species in natural and managed environments). 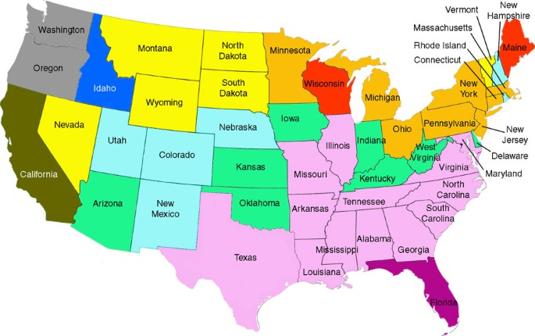Figure 3: US state clustering based on insect pest assemblages. Map of contiguous USA showing those states that were allocated to the same neuron in a SOM analysis (same colour) and hence those states that have the most similar insect pest assemblages. Figure 3: US state clustering based on insect pest assemblages. Map of contiguous USA showing those states that were allocated to the same neuron in a SOM analysis (same colour) and hence those states that have the most similar insect pest assemblages. Full size image The SOM is essentially a statistical approach for predicting likelihood of establishment and identifying the most suitable 'source' locations for pests, but it does not consider the likelihood of a species actually arriving in a state. Therefore, if the SOM model predicts a high likelihood of establishment for a species that is currently absent from a state, it is not possible to determine if the species is absent because it has failed to arrive, or if the SOM prediction is simply inaccurate. However, examining the distribution of absent species across likelihood levels reveals that most absent species from a region occur with the lowest likelihood values, and of those species with high likelihood values, most have already established (see Supplementary Figs S3–S10 for examples). For example, Supplementary Figure S4 shows the distribution of absent species for Alabama. Approximately 97% of the species in the highest likelihood category (0.9–1.0) are present (3% are absent). In the next category (0.8–0.89), approximately 82% of species are present. This trend continues down until the lowest category (0–0.09), where all the species are absent and none are present. This pattern repeats itself in the other examples given in Supplementary Figures S3–S10 and is evidence that the SOM is making appropriate predictions. If species that are present in a state were consistently assigned low likelihood values, this would cast serious doubt over the values generated for absent species. Further validation of the SOM technique can be obtained by comparing our predictions with independent pest distribution data for the United States. The NAPIS pest tracker website ( http://pest.ceris.purdue.edu/pestlist.php ) publishes maps for pests of agricultural and forest commodities based on survey data collected by Cooperative Agricultural Pest Survey and Plant Protection and Quarantine(USDA). These survey maps show, on a county by county basis, where a pest species has or has not been found. We identified 59 insect pest species present in this online database that were also present in the CABI database and compared their observed distributions with the predicted likelihood of establishment from the SOM. Although not a categorical threshold, assuming a likelihood value of 0.5 indicates that the SOM model predicts a species is more likely to be present than absent, we found 86% agreement between observed (from the NAPIS website) and predicted (from the SOM model) species distribution ( Supplementary Data 1 ). These validation results, together with analyses demonstrating that the method is resilient to realistic reporting errors in the species presence/absence [21] , suggest the SOM approach provides a robust method for identifying the invasive species most likely to establish, and the possible source sites based on pest assemblage similarity. The results of our study reveal that, based on a known global list of insect pests, the greatest immediate threats (in terms of establishment likelihood) to the United States come from within, as the majority of pest species most capable of establishing have already established. This is reflected at the state level where, for the majority of states, those species of highest likelihood of establishing can be found in another state, and often a neighbouring state. Although this does not mean that the United States could not be invaded by other recognized pest species, or that new exotic insects cannot arrive and attain pest status, in terms of invasive species policy the results suggest the need for increased awareness of state-level post-border biosecurity [3] , [34] ( http://www.cdfa.ca.gov/phpps/ar/pe_exterior.html ), especially among clustered states, and the possible development of area-wide control strategies to attenuate potential pest spread [35] . Data Data were extracted with permission from the CABI Crop Protection Compendium [23] . This data set is the presence/absence data of 844 insect pests within 459 geographical regions. These regions are political countries with many of the larger countries, such as the USA, further subdivided into their states or provinces. This compendium database is a global compilation of information on all aspects of plant health and the distributional data are sourced from available literature records ( http://www.cabi.org/compendia/cpc/ ). The result was a 459 × 844 matrix comprising 459 vectors each with 844 elements, where each element of a vector represented the presence (1) or absence (0) of an insect species in a region. SOM model A SOM is an artificial neural network capable of converting high-dimensional data into a two-dimensional map in which data points that are found close together on the map are more similar than those that are further away [36] . The SOM therefore is a clustering method in which similar data points (in multidimensional space) are clustered together in the resultant two-dimensional map. Full details describing a SOM analysis can be obtained from refs 22 , 36 , but essentially, each of the 459 regions occupy a particular point in space of 844 dimensions. Each region's position in this space is determined by the 844-element vector that describes the presence or absence of all 844 insect pests in that region. The SOM projects its 108 neurons into this space through neuron weight vectors. As with the region vectors, these neuron weight vectors are composed of 844 elements. In effect, each SOM neuron occupies a point in the same multidimensional space as the regions, thereby allowing them to 'interact' with the region vectors (see below for further explanation). When the analysis is initiated, each raw data point is assessed and the neuron that is closest to this data point in this multidimensional space is deemed to be the best matching unit (BMU). The neuron weight vector of the BMU is adjusted so that it moves closer to the data point. Because all neurons are connected together similar to a large 'elastic net', the process of one neuron moving exerts a gravitational force that drags other neurons in the SOM with it. With each iteration, the neurons spread out to eventually occupy approximately the same area that the data points occupy in the multidimensional space. When the analysis is complete each data point or region vector will have a BMU that is its closest neuron. Regions that have very similar pest assemblages will be located close together in the multidimensional space and will have the same BMU. Each neuron therefore occupies a point in the multidimensional space that is described by its neuron weight vector. In this study, the neuron weight vector comprises 844 elements with each element having a value between 0 and 1. Each element corresponds to one of the 844 insect species and can be interpreted as a likelihood index or an index of how strongly that species is associated with other species in that neuron and hence the species assemblage of any region associated with that neuron (BMU) [25] . The SOM analysis therefore generates likelihood indices for all species regardless of whether they are present or absent from a particular region and, not surprisingly, those species that are already present in a region will receive a high likelihood index. For the USA, the likelihood list generated is the neuron weight of its BMU. The analysis was performed using Matlab [37] and the SOM Toolbox (version 2.0) developed by the Laboratory of Information and Computer Science Helsinki University of Technology ( http://www.cis.hut.fi/projects/somtoolbox/ ) [38] . Further details of the model are reported in Supplementary Methods . A top 100 likelihood list was generated for the United States as a whole and all 48 contiguous US states (see Supplementary Data 1 ). Regression analyses We obtained state size data (km 2 ) from the US Census Bureau ( http://www.census.gov/population/www/censusdata/density.html ) and used linear regression to determine if there was a significant relationship between the size of the state and the number of absent species in a state's top 100 list. We obtained state latitudinal range from Wikipedia's web page for each individual state and confirmed these values using an atlas [39] . We then took the midpoint in a state's latitudinal range and used linear regression to determine if there was a significant relationship between a state's latitude and the number of absent species in a state's top 100 list. We obtained domestic passenger data from the US Bureau of Transportation Statistics ( http://www.transtats.bts.gov/DL_SelectFields.asp?Table_ID=258 ), T-100 Domestic Market (US Carriers) database (2007 data). We then used asymptotic regression (exponential curve) to determine if there was a significant relationship between the numbers of passengers arriving into a state and the number of absent species in a state's top 100 list. We obtained GSP from the US Department of Commerce, Bureau of Economic Analysis ( http://www.bea.gov/regional/gsp/action.cfm ) and used asymptotic regression (exponential curve) to determine if there was a significant relationship between a state's GSP and the number of absent species in a state's top 100 list. All regression analyses were performed using Genstat [40] and for all tests we used a linear and a non-linear regression (an exponential curve). For significant relationships we took the regression that accounted for the largest percentage of variation. For all regressions, standardized residuals were plotted against fitted values to test for homoscedasticity and a histogram of these residuals was generated to determine normality. Determining host availability To ensure that the reason a species was absent from a state was not because of the absence of an available host plant for that species, we counted only those absent species for which a host plant was present in that state. We obtained plant host lists for every pest species absent from a state and in that state's top 100 list from the CABI Crop Protection Compendium [23] . For each pest species we then determined, from the USDA Plants Database ( http://plants.usda.gov/index.html ), if at least one of these host plants was present in the state in which the pest species was absent from. This would determine if a pest species was able to establish in principle in a state. How to cite this article: Paini, D.R. et al . Threat of invasive pests from within national borders. Nat. Commun. 1:115 doi: 10.1038/ncomms1118 (2010).